REGγ is critical for skin carcinogenesis by modulating the Wnt/β-catenin pathway Here we report that mice deficient for the proteasome activator, REGγ, exhibit a marked resistance to TPA (12-O-tetradecanoyl-phorbol-13-acetate)-induced keratinocyte proliferation, epidermal hyperplasia and onset of papillomas compared with wild-type counterparts. Interestingly, a massive increase of REGγ in skin tissues or cells resulting from TPA induces activation of p38 mitogen-activated protein kinase (MAPK/p38). Blocking p38 MAPK activation prevents REGγ elevation in HaCaT cells with TPA treatment. AP-1, the downstream effector of MAPK/p38, directly binds to the REGγ promoter and activates its transcription in response to TPA stimulation. Furthermore, we find that REGγ activates Wnt/β-catenin signalling by degrading GSK-3β in vitro and in cells, increasing levels of CyclinD1 and c-Myc, the downstream targets of β-catenin. Conversely, MAPK/p38 inactivation or REGγ deletion prevents the increase of cyclinD1 and c-Myc by TPA. This study demonstrates that REGγ acts in skin tumorigenesis mediating MAPK/p38 activation of the Wnt/β-catenin pathway. REGγ (also known as PA28γ, PSME3 and Ki antigen) is a member of the 11S family of proteasome activators of the 20S core proteasome. It can promote the degradation of multiple proteins including p53 and MDM2 in an ubiquitin- and ATP-independent manner [1] , [2] , [3] . Previous studies found that REGγ is overexpressed in numerous cancers including breast, thyroid, lung and liver cancers [4] , [5] , [6] , suggesting a potential role for REGγ in tumorigenesis. Non-melanoma skin cancers comprised basal cell carcinoma and squamous cell carcinoma that are the most common of all human cancers. The phorbol ester TPA is a skin tumour promoter, resulting in activation of protein kinase C (PKC) isotypes by mimicking diacylglycerol (DAG) function [7] . Serial activation of some PKCs induced by TPA is crucial for the initiation and progression of skin tumours [8] . PKC isoforms are known to activate multiple MAPK components including ERK, JNK and p38 (ref. 9 ). Abnormalities in the MAPK pathway play a critical role in the development and progression of skin cancer by targeting AP-1 (cJun and cFos) [10] . In a majority of SCC, Ras GTPase and MAPK cascade are activated [11] , [12] . A previous study found that the Wnt/β-catenin/TCF signalling pathway is constitutively activated in non-melanocytic skin tumours [13] . Moreover, abnormal and nuclear localization of β-catenin have been observed in human skin cancer [14] . C-Myc, a downstream target of β-catenin, can regulate p21 and is involved in Ras-driven epidermal tumorigenesis [15] . Thus, it seems that different signalling pathways may connect to each other, contributing to skin tumorigenesis. However, cross-talk between the MAPK signalling pathway and the Wnt /β-catenin signalling pathway has not been demonstrated during the development of skin cancer. In the present study, we demonstrate that REGγ promotes skin tumour development in a two-stage skin carcinogenesis mouse model. TPA stimulation upregulates expression of REGγ via the MAPK/p38 signalling pathway. Subsequently, overexpressed REGγ activates the β-catenin/Wnt signalling pathway through degradation of GSK-3β, leading to abnormal cell proliferation and concurrent papilloma formation. Skin tumour initiation in REGγ -/- mice is markedly inhibited, suggesting that REGγ is critical for skin tumorigenesis. REGγ is critical for skin tumorigenesis in a mouse model The role of REGγ in skin tumour formation was examined in animals by chemical carcinogenesis. Compared with REGγ +/+ mice that had papillomas as early as 9 weeks after the first TPA application, REGγ −/− mice required at least 15 weeks for tumour induction. On average, REGγ +/+ mice developed 6.6 tumours per mouse with 20 weeks of TPA treatment, whereas REGγ −/− mice developed only 1.1 tumours per mouse (two-tailed Student’s t -test, n =10, P <0.001) ( Fig. 1a,b ). The volume of tumours in REGγ −/− mice was markedly reduced in comparison with that in REGγ +/+ mice (two-tailed Student’s t -test, n =10, P <0.001) ( Fig. 1c ), suggesting that REGγ functions as an oncogenic promoter for papilloma formation in a DMBA/TPA tumour model. 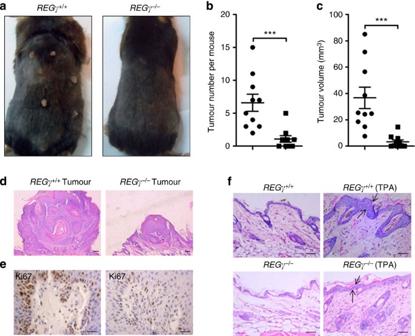Figure 1: REGγ is critical for skin tumorigenesis in a mouse model. (a) Representative photographs of skin tumours showing a protective role of REGγ-deficient mice after 20 weeks of TPA promotion. (b) TPA-induced skin tumour numbers and the mean value per mouse (two-tailed Student’st-test,n=10 for REGγ WT and KO mice, respectively, ***P<0.001). (c) An average tumour volume/mouse (mm3, two-tailed Student’st-test,n=10, ***P<0.001). (d) Representative HE staining of papillomas inREGγWT and KO mice. Scale bar, 100 μm (magnification, × 5). (e) Immunohistochemical staining of Ki67 in papillomas fromREGγWT and KO mice. Scale bar, 25 μm (magnification, × 40). (f) Mouse skin response to a short-term TPA treatment. HE staining of dorsal skin from REGγ WT and KO mice after TPA treatment for four days. Scale bar, 50 μm (magnification, × 20). Figure 1: REGγ is critical for skin tumorigenesis in a mouse model. ( a ) Representative photographs of skin tumours showing a protective role of REGγ-deficient mice after 20 weeks of TPA promotion. ( b ) TPA-induced skin tumour numbers and the mean value per mouse (two-tailed Student’s t -test, n =10 for REGγ WT and KO mice, respectively, *** P <0.001). ( c ) An average tumour volume/mouse (mm 3 , two-tailed Student’s t -test, n =10, *** P <0.001). ( d ) Representative HE staining of papillomas in REGγ WT and KO mice. Scale bar, 100 μm (magnification, × 5). ( e ) Immunohistochemical staining of Ki67 in papillomas from REGγ WT and KO mice. Scale bar, 25 μm (magnification, × 40). ( f ) Mouse skin response to a short-term TPA treatment. HE staining of dorsal skin from REGγ WT and KO mice after TPA treatment for four days. Scale bar, 50 μm (magnification, × 20). Full size image All skin tumours derived from REGγ +/+ and REGγ −/− mice were characterized as well-differentiated squamous cell papillomas ( Fig. 1d ). There were no significant histological differences in tumours from REGγ +/+ and REGγ −/− mice. The number of Ki-67-positive cells in skin tumours from REGγ +/+ mice was higher than that in REGγ −/− mice by immunohistochemistry ( Fig. 1e , Supplementary Fig. 1a ), indicating a tumorigenic potential from action of REGγ. We then examined the effects on epidermal cell proliferation of a single topical treatment of TPA and found that TPA-treated REGγ +/+ mouse skin exhibited a marked increase in epidermal thickness ( Fig. 1f ) along with an increased number of Ki67-positive cells ( Supplementary Fig. 1b,c ), compared with REGγ −/− mice. Thus, the resistance to tumour formation in REGγ-deficient skin is, at least partially, related to decreased proliferation in epidermal cells. These results suggest an early action of REGγ in carcinogenesis. TPA treatment promotes REGγ expression in skin In the TPA-induced mouse cancer and cultured cell models, we found an increased expression of REGγ at mRNA and protein levels ( Fig. 2a–d ). To verify this, we generated a luciferase reporter driven by the REGγ-promoter (REGγ-Luc) and tested TPA-induced expression of this reporter in HaCaT cells. We found that TPA was able to promote REGγ-luciferase activity in HaCaT cells, reflecting that TPA-induced transcription of REGγ is time and dose-dependent ( Fig. 2e,f ). Immunohistochemical data also showed elevated levels of REGγ in TPA-treated skin and TPA-induced tumour tissues compared with those in normal skin ( Supplementary Fig. 2a ), validating the increased expression of REGγ after TPA exposure in skin. Together, these data raise a possibility that REGγ may be a critical factor mediating TPA-induced skin tumour promotion. 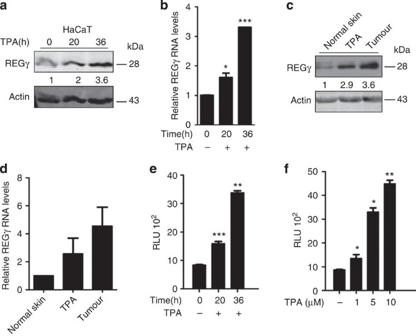Figure 2: TPA promotes expression of REGγin vitroandin vivo. (a) TPA induces REGγ expressionin vitro. HaCaT cells were cultured in the presence or absence of TPA for 20 and 36 h, and REGγ protein levels were examined by western blot. (b) Semi-quantitative RT-PCR analysis of REGγ expression in HaCaT cells following TPA treatment for indicated time (two-tailed Student’st-test,n=3, *P<0.05, ***P<0.001). (c) Immunoblot analysis of REGγ in normal skin, TPA-treated skin and TPA-induced tumour. (d) Semi-quantitative RT-PCR analysis of REGγ expression in samples from (c) (two-tailed Student’st-test,n=3, *P<0.05). (e) HaCaT cells were transfected with a REGγ-promoter luciferase reporter plasmid in the presence or absence of TPA. Cell extracts were analysed in luciferase assays (two-tailed Student’st-test,n=3, **P<0.01, ***P<0.001). (f) Luciferase assays were performed in HaCaT cells after TPA treatment at different concentrations: 0, 1, 5 and 10 μM. (two-tailed Student’st-test,n=3, *P<0.05, **P<0.01). Figure 2: TPA promotes expression of REGγ in vitro and in vivo . ( a ) TPA induces REGγ expression in vitro . HaCaT cells were cultured in the presence or absence of TPA for 20 and 36 h, and REGγ protein levels were examined by western blot. ( b ) Semi-quantitative RT-PCR analysis of REGγ expression in HaCaT cells following TPA treatment for indicated time (two-tailed Student’s t -test, n =3, * P <0.05, *** P <0.001). ( c ) Immunoblot analysis of REGγ in normal skin, TPA-treated skin and TPA-induced tumour. ( d ) Semi-quantitative RT-PCR analysis of REGγ expression in samples from ( c ) (two-tailed Student’s t -test, n =3, * P <0.05). ( e ) HaCaT cells were transfected with a REGγ-promoter luciferase reporter plasmid in the presence or absence of TPA. Cell extracts were analysed in luciferase assays (two-tailed Student’s t -test, n =3, ** P <0.01, *** P <0.001). ( f ) Luciferase assays were performed in HaCaT cells after TPA treatment at different concentrations: 0, 1, 5 and 10 μM. (two-tailed Student’s t -test, n =3, * P <0.05, ** P <0.01). Full size image p38 is essential for TPA-induced overexpression of REGγ It is known that TPA activates MAPK/p38 through multiple PKCs [16] . To address how TPA induced abnormal expression of REGγ, we measured the activities of MAPK pathways. The levels of phosphorylated p38 and cJun were increased in TPA-treated mouse skin compared with untreated controls. More marked elevation of p-p38 and p-cJun was observed in TPA-induced tumours ( Fig. 3a ). It appears the levels of active p38 and cJun are positively correlated with the expression of REGγ ( Fig. 3a ). 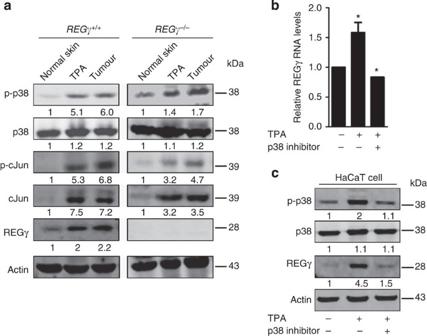Figure 3: p38 MAPK pathway is critical for TPA-induced overexpression of REGγ. (a) Concurrent high expression of active p38, cJun and REGγ in normal skin, TPA-treated skin and TPA-induced tumours fromREGγ+/+andREGγ−/−mice. (b,c) Inhibition of p38 (pre-treated for 1 h) attenuated TPA-induced upregulation of REGγ. Quantitative RT-PCR analysis ofREGγexpression (b) (two-tailed Student’st-test,n=3, *P<0.05) and western blotting results of active p38 and REGγ in HaCaT cells (c) were displayed. Figure 3: p38 MAPK pathway is critical for TPA-induced overexpression of REGγ. ( a ) Concurrent high expression of active p38, cJun and REGγ in normal skin, TPA-treated skin and TPA-induced tumours from REGγ +/+ and REGγ −/− mice. ( b , c ) Inhibition of p38 (pre-treated for 1 h) attenuated TPA-induced upregulation of REGγ. Quantitative RT-PCR analysis of REGγ expression ( b ) (two-tailed Student’s t -test, n =3, * P <0.05) and western blotting results of active p38 and REGγ in HaCaT cells ( c ) were displayed. Full size image To determine whether activation of the MAPK/p38/AP-1 pathway is required for increased REGγ expression in response to TPA, we tested the action of p38 inhibitor, SB202190, on REGγ expression. The specific p38 inhibitor effectively prevented TPA-induced increase of REGγ mRNA and protein expression in HaCaT cells ( Fig. 3b,c ). It is noteworthy that p38 and cJun levels can be enhanced by TPA treatments in the skin of both REGγ +/+ and REGγ −/− mice ( Fig. 3a ), indicating that the MAPK/p38/AP-1 pathway acts upstream of REGγ. However, the activity of JNK (a different MAPK member) was unchanged in the skin before and after TPA treatment ( Supplementary Fig. 2b ), indicating a pathway-specific action by TPA. To address the relation between REGγ and p38/AP-1 signalling pathways, we performed semi-quantitative analysis of these protein levels with IHC staining of human SCC samples. REGγ was highly expressed in 98.2% SCC of tumour samples ( Supplementary Fig. 2c ). Consistently, positive staining of p-cJun was observed in 80% of SCC samples and high levels of p-p38 staining in 84.2% SCC samples ( Supplementary Fig. 2c ). Thus, the expression of REGγ and AP-1 signal molecules was highly correlated in human SCC tumours ( Supplementary Fig. 2c ). Together, these results suggest that the MAPK/p38/AP-1 pathway may be responsible for TPA-induced regulation of REGγ transcription. AP-1 promotes REGγ transcription by binding to its promoter To define which regulatory region(s) in the REGγ promoter is required for transcriptional response to TPA, we generated a series of deletion mutants in the promoter region of the REGγ-Luc construct. Since the (−700/−500) regions had minimal REGγ-Luc activity compared with the −1,300/−1,100 region, the REGγ UTR regions between −1,100 and −900 should contain an element responsive to TPA ( Fig. 4a ). The fact that AP-1 binds to TPA response element (TGACTCA) within target genes [17] facilitated our finding a TPA response element (TRE) in the REG γ gene (−997/−991). A TRE-deleted REGγ-Luc construct was generated and expression of this construct in HaCaT cells had no response to TPA treatment ( Fig. 4b ), suggesting that AP-1 could be a critical regulator for REGγ transcription. 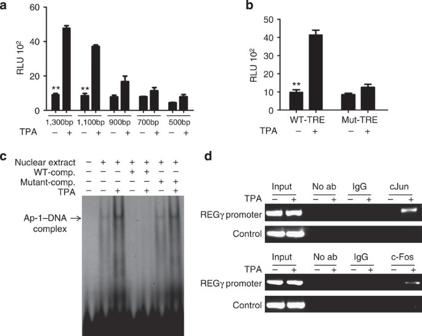Figure 4: Ap-1 directly activates REGγ transcription. (a) Analysis of TPA-responsive regions in the REGγ gene promoter. HaCaT cells were transfected with different deletion constructs of REGγ-Luc reporter in the presence or absence of TPA, and the cell extracts were applied for luciferase assay (two-way ANOVA,n=3, **P<0.01). (b) The TRE in the 5′-UTR ofREGγgene is responsive to TPA induction. HaCaT cells were transfected with a REGγ-Luc reporter or a mutant REGγ-Luc reporter with TRE deletion in the presence or absence of TPA for 24 h followed by luciferase assays. (two-way ANOVA,n=3, **P<0.01). (c) AP-1 directly binds to the TRE-containing DNA sequencein vitro. HaCaT cells were treated with TPA for 24 h, and EMSA assays were performed with the double-stranded oligonucleotides containing a TRE upstream the REGγ promoter. (d) Recruitment of AP-1 to the REGγ promoter region in the genome. CHIP assays were performed with HaCaT cells treated with TPA and antibodies against cJun and c-Fos. Figure 4: Ap-1 directly activates REGγ transcription. ( a ) Analysis of TPA-responsive regions in the REGγ gene promoter. HaCaT cells were transfected with different deletion constructs of REGγ-Luc reporter in the presence or absence of TPA, and the cell extracts were applied for luciferase assay (two-way ANOVA, n =3, ** P <0.01). ( b ) The TRE in the 5′-UTR of REGγ gene is responsive to TPA induction. HaCaT cells were transfected with a REGγ-Luc reporter or a mutant REGγ-Luc reporter with TRE deletion in the presence or absence of TPA for 24 h followed by luciferase assays. (two-way ANOVA, n =3, ** P <0.01). ( c ) AP-1 directly binds to the TRE-containing DNA sequence in vitro . HaCaT cells were treated with TPA for 24 h, and EMSA assays were performed with the double-stranded oligonucleotides containing a TRE upstream the REGγ promoter. ( d ) Recruitment of AP-1 to the REGγ promoter region in the genome. CHIP assays were performed with HaCaT cells treated with TPA and antibodies against cJun and c-Fos. Full size image To elucidate AP-1-mediated regulation of REGγ, EMSA was performed using a TRE probe and HaCaT cell extracts with or without TPA stimulation. We found increased binding of the TRE probe to AP-1 in lysates from cells treated with TPA, indicating that AP-1 is a transcription factor binding to the TRE in REGγ . In the EMSA competition experiments, AP-1 association with the TRE probe was effectively competed by oligonucleotides with intact TRE sequence, but not by mutant oligonucleotides ( Fig. 4c ). Importantly, silencing p38 expression or application of p38 inhibitor blocked AP-1 binding to REGγ promoter ( Supplementary Fig. 3a,b ). To address whether AP-1 acts on the transcription of REGγ in response to TPA in the cell, we performed CHIP assay using primers flanking the TRE in the 5′-UTR of REGγ . As expected, we found that both cJun and c-Fos were recruited to the corresponding region in the CHIP analysis ( Fig. 4d ). Taken together, these results indicate that TPA treatment enhances the activity of AP-1, which directly upregulates REGγ transcription in skin cells. REGγ potentiates Wnt signalling via degradation of GSK-3β To understand how REGγ overexpression leads to skin carcinogenesis following TPA induction, we evaluated the Wnt signalling pathway that has been suggested to play an important role in the progression of skin cancers. We found higher levels of β-catenin in the skin tumour of REGγ +/+ mice than in REGγ −/− mice by western blot and immunohistochemical analysis ( Fig. 5a,b ). Consistently, expression of β-catenin target genes, including CyclinD1 and c-Myc, was increased in REGγ +/+ skin but lowered or had no change in REGγ −/− skin cells ( Fig. 5a,b ). Furthermore, we observed a significant increase in β-catenin, CyclinD1 and c-Myc in REGγ +/+ skin cells treated with TPA ( Supplementary Fig. 3c ). Importantly, both IHC and Western blot data showed an inverse correlation between GSK-3β and β-catenin levels in skin tumour samples from REGγ +/+ and REGγ −/− mice ( Fig. 5a,b ). Taken together, these results demonstrate that REGγ promotes Wnt/β-catenin signalling and enhances the expression of Wnt target genes. 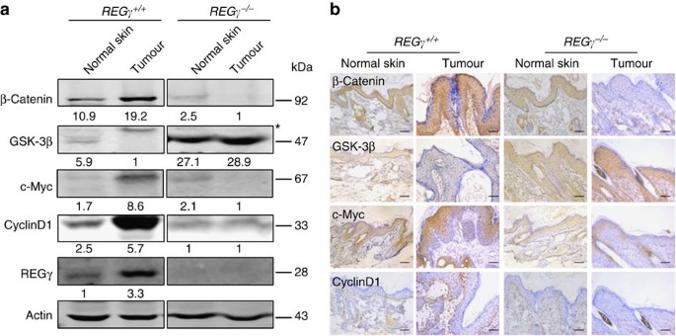Figure 5: REGγ deficiency attenuates the Wnt/β-catenin signalling pathway during skin tumour development. (a) Attenuated expression of Wnt/β-catenin effectors inREGγ−/−skin tumours. Immunoblot analysis of β-catenin, GSK-3β, c-Myc, CyclinD1 and REGγ expression in the normal skin and TPA-induced tumours fromREGγ+/+andREGγ−/−mice. An anti-β-actin immunoblot is shown as the loading controls. Asterisk (*) refers to non-specific bands. (b) IHC analysis of β-catenin, GSK-3β, c-Myc, CyclinD1 in the normal skin and TPA-induced skin tumours fromREGγ+/+andREGγ−/−mice. Scale bar, 50 μm (magnification, × 20). Figure 5: REGγ deficiency attenuates the Wnt/β-catenin signalling pathway during skin tumour development. ( a ) Attenuated expression of Wnt/β-catenin effectors in REGγ −/− skin tumours. Immunoblot analysis of β-catenin, GSK-3β, c-Myc, CyclinD1 and REGγ expression in the normal skin and TPA-induced tumours from REGγ +/+ and REGγ −/− mice. An anti-β-actin immunoblot is shown as the loading controls. Asterisk (*) refers to non-specific bands. ( b ) IHC analysis of β-catenin, GSK-3β, c-Myc, CyclinD1 in the normal skin and TPA-induced skin tumours from REGγ +/+ and REGγ −/− mice. Scale bar, 50 μm (magnification, × 20). Full size image As GSK-3β is required for phosphorylation and subsequent degradation of β-catenin, we tested whether REGγ may directly regulate the stability of GSK-3β. Strikingly, the level of GSK-3β in the skin of REGγ −/− mice was much higher than that in REGγ +/+ mice ( Fig. 6a ). We found no differences in the mRNA level of GSK-3β between REGγ KO and WT skins ( Fig. 6b ). Furthermore, we found physical interactions between REGγ and GSK-3β as defined by a co-immunoprecipitation assay following transient expression of FLAG-REGγ and GSK-3β, alone or in combination with a control vector in 293T cells ( Fig. 6c ). Importantly, co-immunoprecipitation assays using lysates from HaCaT cells demonstrated clear interaction between endogenous REGγ and GSK-3β ( Fig. 6d ). These results suggest that GSK-3β is a target of the REGγ proteasome. 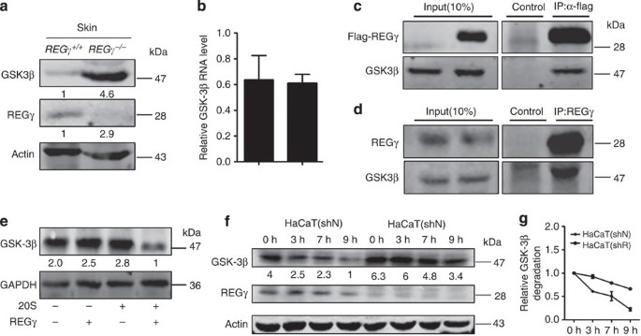Figure 6: REGγ mediates ubiquitin-independent degradation of GSK-3β. (a) REGγ deficiency resulted in GSK-3β elevation in normal skin fromREGγ+/+andREGγ−/−mice. (b) Depletion of REGγ had no effects on the expression of GSK-3β mRNA. (c) REGγ interacts with GSK-3β. Interaction between REGγ and GSK-3β in 293T cells was determined by co-immunoprecipitation and western blot analysis following transient expression of 4 μg of FLAG- REGγ, 2 μg GSK-3β or 4 μg of a FLAG control vector in 293T cells. (d) Co-immunoprecipitation of endogenous REGγ by anti-GSK-3β using lysates from HaCaT cells. (e) REGγ degrades GSK-3βin vitro. Purified REGγ, 20S proteasome andin vitrotranslated GSK-3β were incubated with 20S proteasome at 37 °C for 3 h. An anti-GADPH immunoblot is shown as the loading controls. (f) Silencing REGγ slowed down degradation of endogenous GSK-3β. HaCaT-shN and HaCaT-shR cells were treated with CHX (100 μg ml−1) for indicated times followed by western blotting. (g) Quantitated results in (f) were plotted against indicated time periods to indicate dynamic changes (two-tailed Student’st-test,n=3). Figure 6: REGγ mediates ubiquitin-independent degradation of GSK-3β. ( a ) REGγ deficiency resulted in GSK-3β elevation in normal skin from REGγ +/+ and REGγ −/− mice. ( b ) Depletion of REGγ had no effects on the expression of GSK-3β mRNA. ( c ) REGγ interacts with GSK-3β. Interaction between REGγ and GSK-3β in 293T cells was determined by co-immunoprecipitation and western blot analysis following transient expression of 4 μg of FLAG- REGγ, 2 μg GSK-3β or 4 μg of a FLAG control vector in 293T cells. ( d ) Co-immunoprecipitation of endogenous REGγ by anti-GSK-3β using lysates from HaCaT cells. ( e ) REGγ degrades GSK-3β in vitro . Purified REGγ, 20S proteasome and in vitro translated GSK-3β were incubated with 20S proteasome at 37 °C for 3 h. An anti-GADPH immunoblot is shown as the loading controls. ( f ) Silencing REGγ slowed down degradation of endogenous GSK-3β. HaCaT-shN and HaCaT-shR cells were treated with CHX (100 μg ml −1 ) for indicated times followed by western blotting. ( g ) Quantitated results in ( f ) were plotted against indicated time periods to indicate dynamic changes (two-tailed Student’s t -test, n =3). Full size image To gain additional insight into the mechanism of REGγ-mediated GSK-3β degradation, we examined the capacity of REGγ to direct cell-free proteolysis [18] . Incubation of purified GSK-3β with latent 20S proteasome or REGγ alone exhibited no significant degradation of GSK-3β. However, a combination of REGγ and 20S proteasome promoted marked degradation of GSK-3β ( Fig. 6e ). The half-life of GSK-3β in HaCaT-ShN cells was obviously shorter than that in HaCaT-ShR cells, indicating a faster degradation of GSK-3β in the presence of REGγ ( Fig. 6f,g ). Using cells inducibly expressing a WT REGγ or an enzymatically inactive mutant (N151Y) REGγ, we demonstrated that only cells expressing functional REGγ could repress GSK-3β expression. (Supplementary Fig. 3d). Therefore, we conclude that GSK-3β is a direct target of the REGγ proteasome. REGγ bridges the signalling relays from MAPK to Wnt pathways Next, we tested whether the MAPK/p38/AP-1 pathway could positively modulate the canonical Wnt signalling pathway by controlling REGγ. Intriguingly, we found concurrent increases in p-p38, p-cJun, REGγ, β-catenin, c-Myc and CyclinD1 in TPA-treated WT mouse skin and skin tumours ( Fig. 7a ), but not in a mouse deficient for REGγ ( Supplementary Fig. 4a ). In REGγ −/− skin, p-p38 and p-cJun were increased while β-catenin and its target genes were not elevated ( Supplementary Fig. 4a ). We also observed that expression of REGγ, β-catenin, c-Myc and CyclinD1 were significantly reduced when p38 activity was inhibited ( Supplementary Fig. 3c ). Silencing cJun or p38 by a si-RNA significantly reduced the expression of REGγ, β-catenin, c-Myc and CyclinD1 ( Supplementary Fig. 4b–d ), indicating a regulatory pathway linking AP-1, REGγ and Wnt/β-catenin downstream effectors. Interestingly, the reduction of REGγ, β-catenin, c-Myc and CyclinD1 in the cJun-knockdown cells was effectively restored with overexpression of REGγ ( Supplementary Fig. 5a ). In a mouse xenograft model, tumours derived from REGγ-knockdown A549 cells were significantly smaller than those from A549 cells with normal REGγ expression. Cells expressing a constitutively active β-catenin (S37Y mutant [19] ) can ‘rescue’ REGγ depletion and produce much larger tumours than REGγ knockdown alone ( Fig. 7b , Supplementary Fig. 5b ). Similar results were observed for HaCaT cells ( Fig. 7c , Supplementary Fig. 5c,d ). MTT assay showed that HaCaT cells expressing the active β-catenin proliferated faster than normal cells ( Supplementary Fig. 5e ). Furthermore, we found that REGγ, p-p38 and p-cJun were highly expressed in some human skin tumours compared with normal skin controls ( Fig. 7d , Supplementary Fig. 2c ). In contrast, GSK-3β exhibited a much lower expression level in human skin SCC tumours than in normal skin samples ( Fig. 7d ). Quantified analysis of IHC for human SCC tumours showed REGγ was positively correlated to p-cJun and β-catenin but negatively associated with GSK-3β ( Supplementary Fig. 2c ). Taken together, out data show that REGγ has a novel action, bridging the MAPK/p38/AP-1 pathway and the Wnt/β-catenin pathway in skin tumorigenesis. 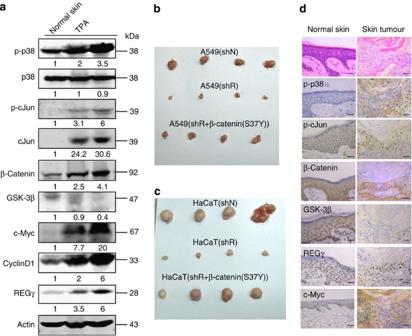Figure 7: REGγ bridges the MAPK/p38/AP-1 pathway and Wnt/β-catenin pathway in skin cancer development. (a) Activation of p38 correlates with overexpression of REGγ and Wnt/β-catenin effectors in the normal skin, TPA-treated skin and TPA-induced tumour. (b) Inhibition of tumour growth by REGγ depletion can be reverted on expression of a constitutively active β-catenin (S37Y) mutated protein. Xenograft tumours were generated by injecting A549(ShN), A549(ShR) and A549(ShR+ β-catenin(S37Y)) cells into dorsal flanking sites. (c) Generation of β-catenin (S37Y) cell lines in HaCaT (ShR) and xenograft tumours as indicated in (b). (d) REGγ is positively correlated with MAPK and Wnt/β-catenin activation in human skin cancers. Representative HE & IHC results showing immunostaining of p-p38, p-cJun, REGγ, β-catenin, GSK-3β and CyclinD1 in human skin cancers and adjacent normal skin controls. Scale bar, 50 μm (magnification, × 20). Figure 7: REGγ bridges the MAPK/p38/AP-1 pathway and Wnt/β-catenin pathway in skin cancer development. ( a ) Activation of p38 correlates with overexpression of REGγ and Wnt/β-catenin effectors in the normal skin, TPA-treated skin and TPA-induced tumour. ( b ) Inhibition of tumour growth by REGγ depletion can be reverted on expression of a constitutively active β-catenin (S37Y) mutated protein. Xenograft tumours were generated by injecting A549(ShN), A549(ShR) and A549(ShR+ β-catenin(S37Y)) cells into dorsal flanking sites. ( c ) Generation of β-catenin (S37Y) cell lines in HaCaT (ShR) and xenograft tumours as indicated in ( b ). ( d ) REGγ is positively correlated with MAPK and Wnt/β-catenin activation in human skin cancers. Representative HE & IHC results showing immunostaining of p-p38, p-cJun, REGγ, β-catenin, GSK-3β and CyclinD1 in human skin cancers and adjacent normal skin controls. Scale bar, 50 μm (magnification, × 20). Full size image In the present study, we analysed the potential role of REGγ in mouse skin carcinogenesis using WT and REGγ −/− model. We demonstrate that REGγ functions as an oncogene for skin tumorigenesis in a two-stage skin carcinogenesis model, in which TPA-induced overexpression of REGγ is dependent on the activation of MAPK/p38 signalling pathway. AP-1 complex can bind directly to the TRE upstream the REGγ promoter and enhance REGγ transcription, ultimately activating the Wnt/β-catenin signalling pathway by augmenting the degradation of GSK-3β. Notably, REGγ acts as a critical factor bridging the MAPK/p38 and the Wnt/β-catenin signalling pathways during skin carcinogenesis, indicating that targeting REGγ could be an alternative approach for skin cancer therapy. As TPA can substitute for naturally occurring diacylglycerol (DAG) for an effective activation of PKC, it is used as a classical skin tumour promoter [20] . PKCs have been implicated as mediators for MAPK/p38 activation [21] , [22] . In addition to mediating TPA-induced skin cancer, p38 is also critical for UV-induced skin carcinogenesis [17] , [23] , [24] . Mice deficient for p38δ exhibit a marked resistance to TPA-induced skin tumour development by impairing ERK1/2-AP-1 and STAT3 pathways [25] . A previous study reported that AP-1-induced involucrin gene expression may be one mechanism in skin tumour development [9] . In this study, we demonstrate that p38 activation is required for REGγ-mediated signalling relays and skin carcinogenesis. Increased transcription of REGγ via the p38/AP-1 signalling pathway reveals an additional mechanism that significantly contributes to the activation of the Wnt/β-catenin signalling and skin tumorigenesis. Despite a positive correlation between MAPK/p38 activation and REGγ overexpression, JNK activation is not observed following TPA stimulation in our study, indicating some specificity in the transduction of TPA-induced carcinogenic signals [26] . A similar phenomenon has been reported; MMP-1 upregulation and TIMP-1 downregulation are p38 (but not ERK or JNK) MAPK-dependent [27] . This is the first study demonstrating that the MAPK/p38 signalling pathway is involved in the regulation of REGγ expression. Interestingly, both Wnt and MAPK/p38 signalling pathways are involved in carcinogenesis and tumour progression, yet possible synergistic contribution to skin cancer is unknown. In the past several years, the cross-talk between the p38/MAPK and the Wnt/β-catenin signalling pathways have been noticed [28] , [29] , [30] with little mechanistic explanation. In this study, we show for the first time that the MAPK/p38/Ap-1 signalling pathway is coupled with the Wnt/β-catenin signalling via the REGγ proteasome system, promoting skin tumour development. This conclusion is also endorsed by our studies using human skin cancer samples. β-Catenin stabilization is involved in upregulation of PKC activity, reflecting a feedback regulation between these two pathways [31] . This may explain our observation that activation of MAPK/p38/AP-1 is stronger in WT than that in REGγ −/− skin after days of TPA treatment ( Fig. 3a ). It is worth emphasizing that REGγ -KO mice also develop a few tumours after 20 weeks of TPA treatments, but with delayed onset, in agreement with the importance of MAPK/p38 signalling for additional targets, such as Stat3, AKT and NFκB [32] . Indeed, combined inhibition of p38 and AKT signalling pathways abrogates cyclosporine A-mediated pathogenesis of aggressive skin SCCs [33] . Thus, additional studies are necessary to elucidate the cross-talk between the p38/MAPK signalling pathway and other signalling molecules during skin carcinogenesis in REGγ -deficient mice. Given that phosphorylation of β-catenin by GSK-3β triggers β-TrCP-mediated degradation of β-catenin [34] , we tested whether REGγ might regulate components in the Wnt/β-catenin pathway. REGγ can directly interact with GSK-3β and promote the degradation of GSK-3β in a ubiquitin-independent manner. Thus, the activation of Wnt/β-catenin signalling pathway followed by REGγ overexpression is dependent on the proteolysis of GSK-3β. Interestingly, we found REGγ deficiency had more profound effects on β-catenin upregulation than on GSK-3β in some experiments. As CK1 is a priming kinase to synergize with GSK-3β for β-TRCP-mediated destruction of β-catenin [35] , our previous finding that REGγ can interact with CK1 and promoted its degradation [21] may interpret this phenomenon. We have shown that REGγ can promote the degradation of cancer suppressor p53 and p21 and thus is likely involved in the regulation of cell cycle and cell growth [2] , [36] . Although p21 is a regulator in skin cancer development [15] , [37] , no striking differences were found in the expression of p53 and p21 between the REGγ +/+ and REGγ −/− skin ( Supplementary Fig. 6a ). In addition, TPA treatment could induce p53 expression in skin of both REGγ +/+ and REGγ −/− mice ( Supplementary Fig. 6b ), indicating that p53 and p21 might be less important factors in the TPA-induced skin cancer model. Whether REGγ-dependent regulation of p53 and p21 occurs in subsets of skin cell types in response to environmental changes deserves further investigation. In summary, our data support a model in which TPA stimulation upregulates the expression of REGγ through the MAPK/p38/AP-1 signal pathway. Overexpressed REGγ degrades GSK-3β and activates the Wnt/β-catenin signalling pathway, leading to an increase in CyclinD1 and c-Myc expression. Conversely, REGγ deletion blocks the linkage between the MAPK/p38/AP-1 signalling and the Wnt/β-catenin signal pathways in response to TPA, attenuating tumour formation ( Fig. 8 ). Thus, REGγ acts as a critical molecule bridging the MAPK/p38/AP-1 pathway and the Wnt/β-catenin pathway during the development of skin carcinogenesis. 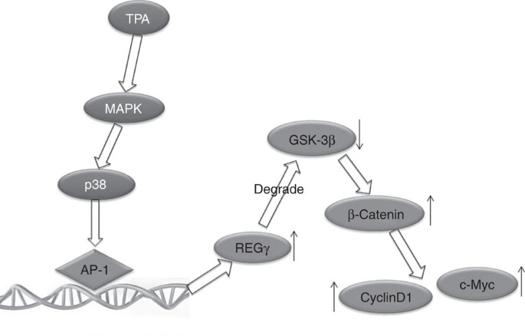Figure 8: A proposed model for the role of REGγ in skin carcinogenesis. In response to TPA, activation of the MAPK/p38/AP-1 signalling pathway stimulates overexpression of REGγ which promotes the degradation of GSK-3β, leading to accumulation of β-catenin and activation of Wnt/β-catenin signalling pathway. Overexpression of proliferation-related genes contributes to, at least in part, abnormal proliferation of keratinocytes and skin tumour development. REGγ acts as an oncogene in skin carcinogenesis by linking the MAPK/p38/AP-1 signalling pathway with the Wnt/β-catenin signalling pathway. Figure 8: A proposed model for the role of REGγ in skin carcinogenesis. In response to TPA, activation of the MAPK/p38/AP-1 signalling pathway stimulates overexpression of REGγ which promotes the degradation of GSK-3β, leading to accumulation of β-catenin and activation of Wnt/β-catenin signalling pathway. Overexpression of proliferation-related genes contributes to, at least in part, abnormal proliferation of keratinocytes and skin tumour development. REGγ acts as an oncogene in skin carcinogenesis by linking the MAPK/p38/AP-1 signalling pathway with the Wnt/β-catenin signalling pathway. Full size image Reagents Antibodies were purchased from Invitrogen (REGγ/PA28γ), BD Pharmingen (p21Cip/WAF1), Sigma (β-actin), Proteintech (GSK-3β, GAPDH), Santa Cruz (cJun, p53), Cell Signaling (p-p38, p-cJun) and Epitomics(β-catenin, c-Myc, CyclinD1). Cycloheximide was purchased from Amresco (Solon, OH). Cell culture and treatment HaCaT cells were purchased from ATCC. The HaCaT stable cell lines were generated by integration of retroviral shRNA vectors specific for REGγ or a control gene (GFP) from OriGene (Rockville, MD). The 293-REGγ-inducible cell line was previously reported [2] . All cell lines were cultured in DMEM supplemented with 10% fetal bovine serum (Gibco). TPA dissolved in acetone at 0.5 μg ml −1 was added to HaCaT cells culture media at a final concentration of 50 ng ml −1 . An MAPK/p38 inhibitor SB202190 dissolved in DMSO was added to the culture media (10 μM) 1 h before TPA treatment. Mice REGγ −/− mice with C57BL/6 genetic background were acquired from Dr John J. Monaco [38] and bred in the Animal Core Facility following procedures approved by the Institutional Animal Care and Use Committee. Genotyping of REGγ +/+ and REGγ −/− mice was carried out by PCR analysis of genomic DNA as described previously [16] . DMBA/TPA treatment All animal experiments were performed with 8-week-old female REGγ +/+ and REGγ −/− mice. Skin tumours were generated as described [39] , [40] , with a single dose of DMBA (50 μg per 100 μl acetone; Sigma-Aldrich) for the first week followed by repetitive TPA applications (6.25 μg per 100 μl acetone; Sigma-Aldrich) every 48 h for 20 weeks. Tumours were assessed weekly and mice were killed 20 weeks after the final treatment. RNA interference and RNA analyses The siRNA against cJun#1 and #2 and p38 shown as follows were described previously [41] , [42] , [43] . Si-cJun 1# 5′-GGAAGCUGGAGAGAAUCGCTT-3′; si-cJun 2# : 5′-GGCACAGCUUAAACAGAAATT-3′; si-p38: 5′-AUGAAUGAUGGACUGAAAUGGUCUG-3′.Tissues and cells were homogenized in 1 ml RNAisoTM Plus lysis buffer (TAKARA). Total RNA was extracted and 2 μg RNA was transcribed into cDNA with M-MLV reverse transcriptase (Invitrogen) following the manufacturer’s instruction. The gene-specific primers are as follows: REGγ sense primer, 5′-ACAAGTGAGGCAGAAGAC-3′; REGγ antisense primer, 5′-ATCATGGCTATTGGTGAG-3′; GSK-3β sense primer, 5′-ATAGAATTCATGTCAGGGCGGCCCAGAACCAC-3′; GSK-3β antisense primer, 5′-CCGCTCGAGTCAGGTGGAGTTGGAAGCTGATG-3′; β-actin sense primer, 5′-CGTCATACTCCTGCTTGCTG-3′; β-actin antisense primer, 5′-GTACGCCAACACAGTGCTG-3′. Western blot analysis and in vitro proteolytic analysis Western blot analysis of proteins extracted from cells was performed as described [2] . Equivalent amounts of total protein from each sample were loaded and immuneblots were analysed using primary antibodies specific for REGγ, p21, p53, GSK-3β, p-p38, p-cJun, p-c-Fos, p38, cJun, β-catenin, c-Myc, GAPDH and CyclinD1 (1:1,000 dilutions) overnight at 4 °C. After incubation with a fluorescent-labelled secondary antibody (1:5,000 dilutions), specific signals for proteins were visualized by a LI-COR Odyssey Infrared Imaging System. In vitro proteolytic analysis was performed using 10 μl of purified GSK-3β, 0.25 μg of purified 20S proteasome and 1 μg of REGγ heptamers for the indicated times in 50 μl reaction volume at 30 °C. An aliquot of the reaction was analysed by western blotting ( Supplementary Figs 7,8 ). Immunohistochemistry and H&E staining Tumours or normal skin samples were fixed with 4% paraformaldehyde for 3 days and were then dehydrated through a graded series of ethanol and embedded in paraffin. Four-μm sections were cut in a microtome (Leica, Germany) and then stained with haematoxylin-eosin (H&E). For immunostaining, slides were heated in a microwave oven at 92 °C for 20 m in a citrate buffer. The samples were then incubated overnight at 4 °C with the primary antibodies at 1:250. Subsequently, they were incubated for 1 h with biotinylated goat anti-rabbit antibody IgG and then for 30 m with Streptavidin-HRP peroxidase. Colour reaction product was visualized by using diaminobenzidine (DAB)-H 2 O 2 as a substrate for peroxidase. All sections were counterstained with haematoxylin. Luciferase assay After transfection with pGL3-REG-γ luciferase vector or the pGL3-Basic vector, HaCaT cells were lysed in the luciferase cell culture lysis buffer (Promega). Cell lysates were vortexed and then centrifuged in 4 °C at 13,000 g for 2 min. Supernatant was added with the luciferase assay substrate (60–80 ml). Luminescence was measured as relative light units, twice for each lysate, taking the reading of luciferase assay using a LUMIstar OPTIMA (BMG Labtech). Each assay was repeated for at least three times. ChIP assay and electrophoretic mobility shift assay For ChIP experiments, cells treated with or without TPA were collected and lysed in lysis buffer (1% SDS, 10 mM EDTA, protease inhibitors and 50 mM Tris–HCl (pH 8.1)). The lysates were then sonicated to result in DNA fragments of 200–1,000 bp in length. Cellular debris was removed by centrifugation and the lysates were diluted 1:10 in ChIP dilution buffer (0.01% SDS, 1.1% Triton X-100, 1.2 mM EDTA, 16.7 mM NaCl, protease inhibitors and 16.7 mM Tris–HCl (pH 8.1)). The samples were immunoprecipitaed with 5 μl of indicated antibodies (IgG, cjun, c-Fos) overnight at 4 °C with rotation. DNA–protein immunocomplexes were isolated with 60 ml of protein A agarose beads for 2 h at 4 °C. The beads were washed, eluted in 250 ml elution buffer (1% SDS and 100 mM NaHCO 3 ) and crosslinkes were reversed by adding NaCl to a final concentration of 200 mM and incubating overnight at 65 °C. The DNA was recovered by phenol/chloroform/isoamyl alcohol (25/24/1) extractions and precipitated with 0.1 volume of 3 M sodium acetate (pH 5.2) and 2 volumes of ethanol using glycogen as a carrier. PCR amplification of the genomic fragments was performed with specific primers flanking putative binding sites on the REGγ promoter. The PCR products were electrophoresed in agarose gels and visualized by ethidium bromide. ChIP primer sequences are as follows: forward: 5′-CATGTTGAAATACTTGTA-3′; reverse: 5′-TCTTCATGCACCCATTCA-3′. Electrophoretic mobility shift assay was performed as described [44] . The probe for electrophoretic mobility shift assay was labelled with FAM fluorescence. The probe sequences were as follows: WT forward: 5′-ACCTACATATGTGACTCACATATTTCTA-3′, WT reverse: 5′-TAGAAATATGTGAGTCACATATGTAGGT-3′; mutant forward: 5′-ACCTACATATGAGTCCTGCATATTTCTA-3′, mutant reverse: 5′-TAGAAATATGCAGGACTCATATGTAGGT-3′. MTT assay and xenograft animal model MTT assay was performed by seeding cells in a 96-well plate at 2.5 × 10 3 cells per well and were cultured for 36 h. Then cells were incubated with MTT solution at 37 °C for 2 h. Absorbance (490 nm) was measured and analysed. For Xenograft animal models, A549 (ShR) cells or HaCaT (ShR) cells were transfected with pcDNA3.1-β-catenin (S37Y) for 48 h and hygromycin used to screen the monoclonal cells. Female BALB/c nude mice at the age of 5 weeks were prepared. Cells were implanted into the dorsal flanking sites of nude mice at 2 × 10 6 cells in 100 ml per spot. Four weeks after injection, mice bearing tumours were killed for the assessment of tumour size and immunohistological examination. Data collection and statistical analysis The statistical data were obtained by GraphPad Prism 5.0 software. The intensity of the western blot results was analysed by densitometry using Bio-Rad Quantity One 4.4.0 software. The results were expressed as the mean±s.d. Statistical analysis was performed using two-tailed, paired Student’s t -test or two-way ANOVA. A P value of less than 0.05 was considered statistically significant. How to cite this article: Li, L. et al . REGγ is critical for skin carcinogenesis by modulating the Wnt/β-catenin pathway. Nat. Commun . 6:6875 doi: 10.1038/ncomms7875 (2015).